Characterization and modelling of interspecies electron transfer mechanisms and microbial community dynamics of a syntrophic association Syntrophic associations are central to microbial communities and thus have a fundamental role in the global carbon cycle. Despite biochemical approaches describing the physiological activity of these communities, there has been a lack of a mechanistic understanding of the relationship between complex nutritional and energetic dependencies and their functioning. Here we apply a multi-omic modelling workflow that combines genomic, transcriptomic and physiological data with genome-scale models to investigate dynamics and electron flow mechanisms in the syntrophic association of Geobacter metallireducens and Geobacter sulfurreducens . Genome-scale modelling of direct interspecies electron transfer reveals insights into the energetics of electron transfer mechanisms. While G. sulfurreducens adapts to rapid syntrophic growth by changes at the genomic and transcriptomic level, G. metallireducens responds only at the transcriptomic level. This multi-omic approach enhances our understanding of adaptive responses and factors that shape the evolution of syntrophic communities. Microorganisms in nature do not exist as pure cultures, but rather are involved in a wide variety of interactions and nutritional interdependencies with their bacterial, archaeal and eukaryotic neighbours in their ecosystem. Syntrophy is one such nutritional dependency where two or more microbes combine each other’s metabolic capabilities for the degradation of a particular substrate that neither is capable of performing individually [1] . Syntrophy in which electrons are shared between two partners is central to the functioning of a variety of methanogenic environments such as wetlands, aquatic sediments, animal intestinal systems and oil reservoirs, as well as in anaerobic digesters converting organic wastes to methane [2] , [3] . Furthermore, interspecies electron transfer is considered to have an important role in microbial aggregates that anaerobically oxidize methane with the reduction of sulphate [4] . Traditional biochemical approaches have been able to shed light on the overall physiological activity and mechanisms of electron transfer in many of these microbial communities [5] , [6] . Despite these approaches, it has been challenging to gain comprehensive insights into the dynamics, the factors favouring one mechanism of interspecies electron transfer over the other, as well as genomics features for the metabolic activity of individual constituents. This has necessitated the development of genome-scale approaches that can provide a link between the genotypes of the microbes, their reaction mechanisms and eventually their effect on the functioning of the microbial community [7] , [8] . One of the major goals of microbial ecology and systems biology is to comprehensively understand, characterize and obtain meaningful insights into the various modes of interactions in communities and their functional effect on the ecosystem [9] . Constraint-based modelling approaches (COBRA) using genome-scale metabolic networks have provided significant mechanistic insights into the genotype–phenotype relationship of single bacterial species [10] . Recently, several COBRA methods have been deployed to investigate the various microbial interactions such as mutualism, competition and parasitism [10] , [11] , [12] , [13] , [14] , [15] . One of the first such modelling studies applied flux balance analysis to investigate the mutualism between the sulphate-reducing bacterium Desulfovilbrio vulgaris and the methanogenic archaeon Methanococcus maripaludis [15] . An extension of dynamic flux balance analysis has also been used to characterize the competitive relationship between Geobacter sulfurreducens and Rhodoferax ferrireducens in the subsurface [16] . A COBRA-based computational framework has been applied to determine the media compositions that induce putative symbiotic interactions between all possible combinations of seven different microorganisms [11] . Although this provided the proof-of-concept for integration of multiple genome-scale metabolic models, the nature of the microbial partners evaluated in this study precluded a detailed mechanistic investigation into all possible modes of interactions. Most recently, a general multi-objective optimization framework has been developed for analysing interspecies metabolite transfers during various types of multi-species interactions [13] . Extension of these community systems biology [9] approaches for studying syntrophic associations requires a comprehensive characterization of the various mechanisms of energy transfer and their effect on the functioning of the microbial community. The long-standing paradigm for interspecies electron transfer in methanogenic systems has been interspecies hydrogen transfer, in which the electron-donating partner disposes of electrons by reducing protons to produce hydrogen and the electron-accepting partner accepts electrons by oxidizing hydrogen with the reduction of carbon dioxide to methane [1] . However, direct interspecies electron transfer (DIET) seems to be the primary mode of electron transfer in some methanogenic environments [17] , [18] , [19] . Defined cocultures of Geobacter metallireducens and Geobacter sulfurreducens grow syntrophically via DIET in medium with ethanol as the electron donor and fumarate as the electron acceptor [20] , [21] , [22] and provide a model for syntrophic growth in which both partners are genetically tractable [23] , [24] . Furthermore, a syntrophic coculture in which G. sulfurreducens also operates as the electron-accepting partner, but which functions via interspecies hydrogen transfer, is available for comparison [21] . Here, we expand the scope of community systems biology by developing an integrated modelling framework that combines physiological, transcriptomic and next-generation sequencing data with genome-scale metabolic models to simulate and investigate syntrophic interactions and their associated electron transfer mechanisms. Specifically, we apply this framework to characterize the mechanistic basis of the syntrophic association of G. metallireducens and G. sulfurreducens . By modelling different genetic perturbations of this system, we provide additional insights into the process of DIET, hypothesized to be an important mode of electron transfer in certain syntrophic associations. We further use transcriptomic and genomic data to describe the dynamics of the interaction between the two individual Geobacter species and elucidate their adaptive response to syntrophic growth. Integrated framework for modelling syntrophy and DIET We developed a four-step modelling workflow to enable the genome-scale investigation of metabolic interactions and electron flow in the syntrophic association between G. metallireducens and G. sulfurreducens . First, we developed a protocol to represent the extracellular electron transfer pathways through all the known electron carriers in the cell, including cytochromes, quinone, ferredoxin, NAD and FAD ( Fig. 1a ). In addition to accurately assigning the stoichiometry associated with the respective redox reactions, these pathways also account for thermodynamic consistency, appropriate gene association and cellular localization of the different electron carriers. Second, we implemented this protocol on the genome-scale reconstructions of G. metallireducens and G. sulfurreducens [25] , [26] , [27] to explicitly account for a detailed representation of the energy metabolism involved in extracellular and direct electron transfer. In addition to the updated G. metallireducens model (iAF987) consisting of 987 genes and 1,284 reactions, this step resulted in a model of G. sulfurreducens (iHN837) consisting 837 genes and 1,085 reactions ( Fig. 1b ). Third, to model the metabolic interactions, we integrated these two genome-scale models using an extension of the compartmentalized modelling approach [11] , [12] , [13] . This integrated genome-scale model of syntrophy that consists of 1,824 genes and 2,333 reactions in total, and five compartments, where each species was assumed to have independent cytosol and periplasm compartments. The fifth compartment, the shared metabolite pool (SMP), represents an extracellular environment common to both the constituents ( Fig. 1c ). Fourth, we model DIET by introducing a constraint in the form of a reaction that represents the stoichiometric transfer of electrons between metabolites that correspond to their respective outer membrane cytochromes. Outer membrane cytochromes in Geobacter species have been shown to have a critical role in extracellular electron transfer to minerals as well as other external electron acceptors such as the anode of a microbial fuel cell [28] , [29] . Specifically, the gene encoding OmcS of G. sulfurreducens was shown to be essential for DIET in this syntrophic consortium [20] . Hence, we associated this gene with the reaction representing DIET. We calculated the maximum electron transfer flux through DIET ( ) based on the midpoint potential of OmcS ( Fig. 1d ). This integrated workflow enabled a multi-level characterization of the metabolic interactions and electron flow in the syntrophic association of G. metallireducens and G. sulfurreducens . 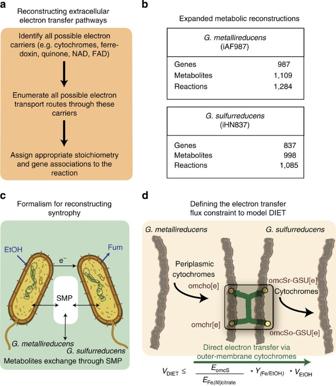Figure 1: Integrated framework for modelling syntrophy and direct electron transfer. (a) Protocol adopted for reconstructing extracellular electron transfer pathways. It must be noted that the exact mechanistic details of extracellular electron transfer remains to be characterized. (b) Properties of the updated and expanded genome-scale metabolic reconstructions used. (c) Formalism for reconstructing syntrophy. Using an extension of the compartmentalized framework, a SMP is included to facilitate exchange of metabolites between the species as well as with the environment. The purple arrows indicate the critical inputs (ethanol oxidation rate and fumarate reduction rate) that are set during each simulation based on physiological data. (d) Defining the electron transfer flux constraint to enable modelling of DIET. The maximum flux through DIET is calculated based on the midpoint potential of OmcS. Figure 1: Integrated framework for modelling syntrophy and direct electron transfer. ( a ) Protocol adopted for reconstructing extracellular electron transfer pathways. It must be noted that the exact mechanistic details of extracellular electron transfer remains to be characterized. ( b ) Properties of the updated and expanded genome-scale metabolic reconstructions used. ( c ) Formalism for reconstructing syntrophy. Using an extension of the compartmentalized framework, a SMP is included to facilitate exchange of metabolites between the species as well as with the environment. The purple arrows indicate the critical inputs (ethanol oxidation rate and fumarate reduction rate) that are set during each simulation based on physiological data. ( d ) Defining the electron transfer flux constraint to enable modelling of DIET. The maximum flux through DIET is calculated based on the midpoint potential of OmcS. Full size image Analysis of carbon and electron flow We employed constraint-based modelling methods to the integrated genome-scale metabolic model to characterize the carbon and electron flow defining the syntrophic association of G. metallireducens and G. sulfurreducens with ethanol and fumarate. We optimized this model with the objective of maximal growth of both constituents ( G. metallireducens and G. sulfurreducens ) with the addition of a constraint for simulating DIET. Specifically, we constrained the electron transfer flux through DIET ( V DIET ) to its maximal value ( ). ( Fig. 1d ). To set the input/output constraints for this simulation, we used experimentally measured physiological uptake rates ( Supplementary Fig. S1 ) and product secretion rates. The ratio of flux through the respective biomass objective functions was used to estimate the relative abundance of the constituents in the community. Model simulations reveal that G. sulfurreducens accounted for 73% of the consortium ( Supplementary Fig. S2 ). This prediction is in accordance with experimental observations of a G. sulfurreducens- dominated coculture with a composition of around 75% G. sulfurreducens [20] . The electron transfer flux through DIET was predicted to be at its maximal value ( ) in this simulation. Further analysis of this optimal flux distribution revealed that G. metallireducens secreted acetate into the SMP as a result of ethanol oxidation. The secreted acetate was predicted to be utilized by G. sulfurreducens as a carbon source for growth. In addition to DIET, acetate was also predicted to serve as an electron donor for fumarate reduction via the TCA cycle in G. sulfurreducens ( Fig. 2 ). To assess the accuracy of these model-predicted flux distributions, we constructed a context-specific model based on transcriptomic profiling of this coculture using the GIMME algorithm [30] . This algorithm implements an optimization framework to determine the model that best describes the gene expression levels and metabolic objectives of the cell under the given conditions. Additionally, the GIMME algorithm outputs a consistency score [30] that quantifies the agreement of metabolic network with expression data. The resulting context-specific model had a consistency score of 0.99 and consisted of 988 reactions and 993 metabolites. Reactions such as citrate synthase (CS) and aconitase of G. metallireducens , formate dehydrogenase and the uptake hydrogenase of G. sulfurreducens , were not active in this context-specific model. This prediction agrees with the demonstration of syntrophic growth between G. metallireducens and a mutant of G. sulfurreducens lacking both the uptake hydrogenase and formate dehydrogenase [21] . In another in silico simulation, where each reaction was knocked out individually to assess their effect on growth, it was revealed that apart from uptake of ions, the main reactions predicted to be essential for sustenance of syntrophic interaction in this consortium are those involved in the ethanol oxidation, fumarate reduction, and DIET ( Supplementary Table S1 ). 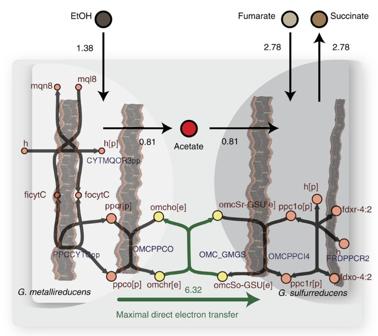Figure 2: Carbon and electron flow in the consortium. Flux distribution in the wild-type syntrophic interaction betweenG. metallireducensandG. sulfurreducens. All flux values are shown in mmol per gram DW per h. The figure shows flux values corresponding to physiologically measured ethanol uptake rate (1.38 mmol per gram DW per h). Reaction abbreviations: CYTMQOR3pp represents electron transfer from menaquinone pool to cytochromes inG. metallireducens; PPCCYTCpp and OMCPPCO represents the electron transfer reactions from the inner membrane cytochromes to theomcSinG. metallireducens; OMC_GMGS is the reaction representing DIET betweenomcSofG. metallireducensandG. sulfurreducens; OMCPPCI and FRDPPCR2 are the reactions corresponding to electron transfer intoG. sulfurreducensto the intracellular reducing equivalents in the form of ferredoxin. Figure 2: Carbon and electron flow in the consortium. Flux distribution in the wild-type syntrophic interaction between G. metallireducens and G. sulfurreducens . All flux values are shown in mmol per gram DW per h. The figure shows flux values corresponding to physiologically measured ethanol uptake rate (1.38 mmol per gram DW per h). Reaction abbreviations: CYTMQOR3pp represents electron transfer from menaquinone pool to cytochromes in G. metallireducens ; PPCCYTCpp and OMCPPCO represents the electron transfer reactions from the inner membrane cytochromes to the omcS in G. metallireducens ; OMC_GMGS is the reaction representing DIET between omcS of G. metallireducens and G. sulfurreducens ; OMCPPCI and FRDPPCR2 are the reactions corresponding to electron transfer into G. sulfurreducens to the intracellular reducing equivalents in the form of ferredoxin. Full size image As both G. metallireducens and G. sulfurreducens are capable of fixing nitrogen, we investigated the impact of this energy intensive process on the syntrophic interaction by simulating syntrophic growth in ammonia-free medium. This analysis predicted that if G. sulfurreducens was to be the organism fixing nitrogen for the community, the composition of the community would consist of at least 45% G. metallireducens . On the other hand, no feasible interaction was predicted if G. metallireducens had to be the organism solely responsible for fixing nitrogen for the community. Further inspection of the flux distribution in the latter scenario reveals that the energy yield is insufficient to meet the ATP requirements for the nitrogenase reaction of G. metallireducens to carry a flux that meets the needs of both interacting partners. This prediction is experimentally validated by the lack of syntrophic growth observed in a coculture of G. sulfurreducens nifD mutant, which is unable to fix nitrogen [23] and a G. metallireducens strain preadapted to fix nitrogen in a medium containing nitrogen gas as the sole nitrogen source ( Supplementary Fig. S3 ). Although this does not address the sufficiency of nitrogen fixation by G. sulfurreducens , the modelling prediction and experimental validation demonstrates that nitrogen fixation by G. sulfurreducens is necessary for this syntrophic interaction. Transcriptomic insights into the mechanisms of electron transfer To gain further insights into the different mechanisms of electron transfer in the consortium, we analysed the transcriptome and modelled two mutant strains of G. sulfurreducens in a coculture with G. metallireducens , where the possibility of acetate oxidation or hydrogen uptake by G. sulfurreducens was eliminated. This was achieved by the deletion of citrate synthase (CS K.O. strain) and the uptake hydrogenase of G. sulfurreducens (hyb K.O. strain) to eliminate acetate oxidation and hydrogen transfer, respectively ( Table 1 ) [22] . Table 1 Details of the different strains modelled. Full size table Although G. metallireducens has not been shown to be capable of generating hydrogen gas [31] under its typical growth conditions, it could be argued that there might be some unidentified gene in G. metallireducens that could be activated only when G. metallireducens is engaged in syntrophic association. It is also known that G. metallireducens could, in principle, generate some hydrogen as a byproduct of the nitrogenase reaction. Specifically to rule out this possibility, we profiled the transcriptome of the hyb K.O. strain. Deleting the uptake hydrogenase of G. sulfurreducens in this consortium resulted in the differential expression of 145 genes in G. sulfurreducens ( Fig. 3a , Supplementary Data 1 ). Specifically, we observed an increased expression (>4-fold) of the outer membrane cytochromes ( omcS, omcT ) that are believed to be involved in DIET and a significant downregulation (>15-fold) in expression of the other hydrogenase ( hya ) in addition to the deleted hyb . Consistent with the lack of hya activity in the context-specific model for the WT strain, the predicted flux distribution for the hyb K.O. strain was similar to that of the WT strain. This similarity was further supported by comparable ethanol and fumarate uptake rates observed in both these strains [22] ( Fig. 3b ). 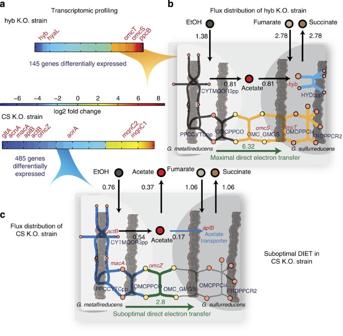Figure 3: Insights into the mechanisms of electron transfer from transcriptomic data. (a) Fold changes observed for the differentially expressed genes in the hyb K.O. strain and CS K.O. strain. (b) Metabolic interpretation of the transcriptomic differences in the hyb K.O. strain relative to the WT strain. The main genes unregulated in the hyb K.O. strain include theomcSthat are associated with the pathway for DIET in the consortium. (c) Metabolic adjustments in the CS K.O. strain based on the transcriptomic data. The elimination of interspecies electron transferviaacetate oxidation confers a suboptimal direct electron transfer phenotype to the consortium. This is mirrored by the significant suppression of the electron transfer pathway involved in DIET inG. metallireducens. All flux values are in mmol per gram DW per h. Figure 3: Insights into the mechanisms of electron transfer from transcriptomic data. ( a ) Fold changes observed for the differentially expressed genes in the hyb K.O. strain and CS K.O. strain. ( b ) Metabolic interpretation of the transcriptomic differences in the hyb K.O. strain relative to the WT strain. The main genes unregulated in the hyb K.O. strain include the omcS that are associated with the pathway for DIET in the consortium. ( c ) Metabolic adjustments in the CS K.O. strain based on the transcriptomic data. The elimination of interspecies electron transfer via acetate oxidation confers a suboptimal direct electron transfer phenotype to the consortium. This is mirrored by the significant suppression of the electron transfer pathway involved in DIET in G. metallireducens . All flux values are in mmol per gram DW per h. Full size image Eliminating the possibility of electron transfer through acetate oxidation (CS K.O. strain) resulted in the differential expression of 485 genes in both G. metallireducens and G. sulfurreducens ( Fig. 3a , Supplementary Data 2 ). One hundred and forty-five genes out of the 485 differentially expressed genes encoded for at least one reaction in the genome-scale model. A statistical analysis on these 145 genes based on the metabolic subsystems revealed a significant enrichment for genes involved in energy metabolism and electron transfer ( P -value 0.01; hypergeometric test). We used experimentally measured physiological uptake rates for the CS K.O. strain to constrain the model and to simulate the effect of the elimination of additional electron transfer via acetate. The optimal ratio of the constituents in this consortium was predicted to be 44% G. metallireducens , which compared well with the experimental observation of about 50%. As expected, 67% acetate secreted by G. metallireducens accumulated in the SMP, due to the inability of G. sulfurreducens to oxidize it. In accordance with this prediction, the expression of acetate transporter genes in G. sulfurreducens decreased significantly (>15-fold) compared with that of the WT strain. Similar to the WT strain, DIET was predicted to be preferred over interspecies hydrogen transfer in the CS K.O. strain. However, the electron transfer flux through DIET in the CS K.O strain occurred at just the 75% maximal value. This suboptimal electron transfer scenario observed in the CS K.O. strain could potentially result in a lower electrical conductivity in this consortium compared with the WT strain. We investigated the metabolic adjustment to this suboptimal electron transfer scenario by integrating the fold changes in gene expression of the two strains with the genome-scale model using MADE [32] . This analysis revealed that the agreement between metabolic adjustments predicted by the model with the transcriptomic profiling was 87% accurate with a significant increase in flux for 17 reactions and decrease in flux for 91 reactions. The reactions showing significant decrease in fluxes corresponded to the electron transfer pathway of G. metallireducens involved in DIET (CYTMQOR3pp_D, NADH17pp_D, OMCPPCO_D) ( Fig. 3c ). The changes in the flux distribution observed from expression data were also further corroborated by the use of randomized Monte Carlo sampling on the genome-scale model. This significant suppression of the critical components of the electron transfer pathway out of G. metallireducens mirrors the suboptimal electron transfer scenario observed upon eliminating the additional electron transfer via acetate ( Fig. 3c ). This integrated analysis of transcriptomic data with genome-scale model of syntrophy reveals a unique interaction motif between the different modes of electron transfer. Acetate transfer was thought to primarily contribute to the extra source of electrons for G. sulfurreducens and thereby contribute to its higher relative abundance in the consortium. However, the conferral of a suboptimal electron transfer scenario in the CS K.O. strain reveals an unexpected effect on the energetic efficiency of DIET in the absence of acetate transfer. This leads us to postulate a potential positive effect on DIET due to acetate transfer. Dynamics of adaptation to syntrophic growth The obligate syntrophic association between the two Geobacter species was achieved through adaptive laboratory evolution under a selection pressure to switch from their Fe(III)-reducing growth mode to rapid syntrophic growth in ethanolfumarate medium. Other members of the Geobacteraceae like Pelobacter carbinolicus , have been previously shown to evolve from an Fe(III) reducer to a syntroph performing interspecies hydrogen transfer [21] , [33] , [34] . In the association described in this study, G. metallireducens functions as an ethanol-oxidizing syntroph performing DIET [20] . On the other hand, the selection pressure dictates G. sulfurreducens to depend on G. metallireducens to derive its carbon source as well as electrons for growth while reducing fumarate. We used the genome-scale model of the consortium to investigate the effect of the selection pressure on the dynamics of adaptation to syntrophic growth. First, we assessed the entire spectrum of feasible interactions in this consortium by evaluating the effect of relative rates of ethanol oxidation and fumarate reduction. This phenotypic phase plane analysis [35] indicated the presence of two distinct feasible phases (Phases A and B) based on the presence or absence of a limitation on fumarate reduction rate. The line of optimality represents the ethanol and fumarate uptake rates that correspond to optimal growth of the consortium ( Fig. 4 ). Phase A is closer to the line of optimality and there is no limitation due to fumarate uptake rate. This phase is also characterized by maximal electron transfer flux through DIET as described by ( ). This state reflects the ideal scenario for both G. metallireducens and G. sulfurreducens in this consortium. Experimentally determined uptake rates of WT aggregates are representative of Phase A, with maximal electron transfer through DIET. Typically, in Phase A, G. sulfurreducens dominates the consortium and is most abundant. Phase B reveals a scenario where a limitation due to fumarate uptake rate results in a state of suboptimal electron transfer flux. The electron transfer flux from G. metallireducens to G. sulfurreducens is limited by the rate of electrons that G. sulfurreducens can transfer to fumarate. Although G. sulfurreducens still derives the requisite amount of electrons to reduce fumarate, G. metallireducens is forced to find other ways to transfer the electrons it derives from ethanol oxidation. An example of the physiological characteristic exhibited in Phase B is the CS K.O. strain, with a relative abundance of G. metallireducens closer to 50%, the inability to oxidize acetate and suboptimal DIET. The dynamics of this phenotypic phase plane suggests that the metabolic capabilities of G. sulfurreducens are more streamlined to meet the selection pressure of rapid syntrophic growth. This could likely be due to an active response at the genomic level. Consistent with this, a 1 bp deletion in GSU1495 encoding PilR of G. sulfurreducens shown to promote syntrophic growth via direct exchange of electrons in cocultures after 100 generations was preserved at the end of 780 generations. Strikingly, even after 780 generations, no genetic mutations were observed in G. metallireducens ( Supplementary Table S2 ). Although G. sulfurreducens undergoes several genomic changes in addition to transcriptomic changes to actively respond to the pressure of rapid syntrophic growth, G. metallireducens responds only at the level of the transcriptome by regulating its expression ( Fig. 3c ). 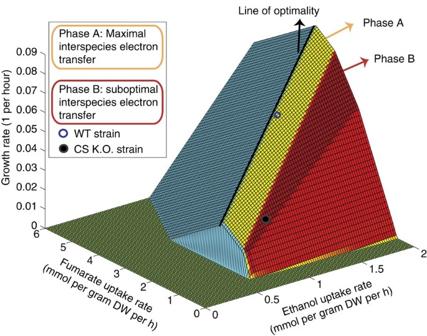Figure 4: Dynamics of interaction between the partners. Phenotypic phase plane analysis reveals the presence of two distinct phases with maximal and suboptimal direct interspecies electron transfer. Figure 4: Dynamics of interaction between the partners. Phenotypic phase plane analysis reveals the presence of two distinct phases with maximal and suboptimal direct interspecies electron transfer. Full size image Comparative analysis of electron transfer mechanisms In contrast to electron exchange via DIET in this system, cocultures of Pelobacter carbinolicus and G. sulfurreducens growing in a similar ethanol/fumarate medium exchange electrons via interspecies hydrogen transfer [21] . This difference can be attributed in part to the inability of P. cabinolicus to make effective electrical connections with extracellular electron acceptors [36] as well as the inability of G. metallireducens to generate hydrogen under growth conditions so far tested [31] . Electron transfer mechanisms are fundamental for syntrophic interactions to exist, and therefore, it is important to assess their influence on the energetic yields of the interacting organisms. Therefore, for an appropriate comparison of the energy yields of the respective partners during the different modes of interspecies electron transfer, we used the coculture of P. carbinolicus and G. sulfurreducens as the system for the hydrogen transfer scenario. We modified the genome-scale metabolic model of G. metallireducens to account for the major differences involved in ethanol and hydrogen metabolism of P. carbinolicus . This modification mainly included the production of hydrogen via electron confurcation due to the addition of a nicotinamide adenine dinucleotide phosphate-dependent hydrogenase and the Nfn complex, the addition of the Rnf complex and the acetylating acetaldehyde dehydrogenase. The phenomenon of electron confurcation has been shown to have an important role in interspecies hydrogen transfer during syntrophic associations [37] . We evaluated the relative efficiency of the different modes of electron transfer using the community models to obtain insights into the potential differences in the energy conservation mechanisms. Specifically, we computed the maximum molar yield of ATP obtained per mole of electron donor (ethanol) for both the partners in each of the different scenarios. The predicted energy yields of the two partners during DIET mirrored the ratio of the relative abundance observed in the CS K.O. strain. The presence of additional electron transfer via acetate enhanced the efficiency of DIET by 24% ( Fig. 5a ). In this case, the predicted relative energy efficiencies of the two partners were consistent with the observed and predicted values of their relative abundances in the WT strain. The energy yield of G. sulfurreducens was predicted to be about 82% of the total energy yield during hydrogen transfer. This prediction is in good agreement with the reported relative abundance of 85% G. sulfurreducens in its syntrophic association with P. carbinolicus [21] . Although the energy yield for the electron-accepting organism ( G. sulfurreducens ) during interspecies hydrogen transfer was of similar order of magnitude compared with DIET (2.7 versus 3.5), the energy yield of the electron-donating organism was about four times lower during the case of interspecies hydrogen transfer ( Fig. 5a ). The metabolic characteristic governing this significant difference was found to be the mode of energy conservation adopted by P. carbinolicus and G. metallireducens during interspecies hydrogen transfer and DIET, respectively. P. carbinolicus was found to primarily generate ATP via substrate-level phosphorylation, whereas G. metallireducens conserved energy via respiration aided by the establishment of a proton gradient during DIET ( Supplementary Fig. S4 ). This mechanistic difference potentially explains the higher relative abundance of the electron-accepting organism during interspecies hydrogen transfer as observed in the coculture of P. carbinolicus and G. sulfurreducens [21] . 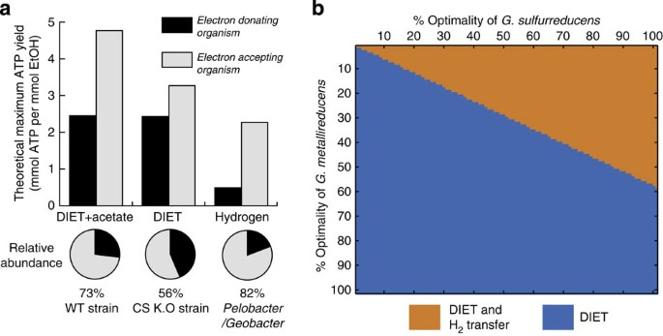Figure 5: Comparing interspecies electron transfer mechanisms. (a) Relative efficiency of the different modes of interspecies electron transfer. DIET+acetate case represents the WT strain, DIET case represents the CS K.O. strain and the hydrogen transfer case is simulated using the cocultureP. carbinolicusandG. sulfurreducens. The maximum energy yield per mol of electron donor is calculated for each mode of interspecies electron transfer. The theoretical maximum for the net reaction in this consortium is 8.27. The pie charts represent the relative abundance of the interacting partners during each mode of interspecies electron transfer. (b) Relationship between community dynamics and mode of interspecies electron transfer. Simulations were carried out with a community model capable of doing hydrogen transfer and DIET. Simulations were conducted over the entire range of optimality levels of both the interacting organisms and whether DIET or hydrogen transfer occurred was monitored. The blue area represents the sole occurrence of DIET during the interaction and the orange area shows the region where DIET and hydrogen transfer occur. Interspecies hydrogen transfer occurred in addition to DIET, in regions where the optimality levels of the electron-accepting organism was at least 1.8 times that of the electron-donating organism. Figure 5: Comparing interspecies electron transfer mechanisms. ( a ) Relative efficiency of the different modes of interspecies electron transfer. DIET+acetate case represents the WT strain, DIET case represents the CS K.O. strain and the hydrogen transfer case is simulated using the coculture P. carbinolicus and G. sulfurreducens . The maximum energy yield per mol of electron donor is calculated for each mode of interspecies electron transfer. The theoretical maximum for the net reaction in this consortium is 8.27. The pie charts represent the relative abundance of the interacting partners during each mode of interspecies electron transfer. ( b ) Relationship between community dynamics and mode of interspecies electron transfer. Simulations were carried out with a community model capable of doing hydrogen transfer and DIET. Simulations were conducted over the entire range of optimality levels of both the interacting organisms and whether DIET or hydrogen transfer occurred was monitored. The blue area represents the sole occurrence of DIET during the interaction and the orange area shows the region where DIET and hydrogen transfer occur. Interspecies hydrogen transfer occurred in addition to DIET, in regions where the optimality levels of the electron-accepting organism was at least 1.8 times that of the electron-donating organism. Full size image The biochemical constraints that govern microbial communities often result in constituents operating at varying levels of optimality that compromises their respective growth objectives [38] . To assess the preferential occurrence of DIET or interspecies hydrogen transfer, we scanned the entire spectrum of optimality for both the electron-donating and electron-accepting organisms using the genome-scale model of syntrophy with the added capabilities of interspecies hydrogen transfer. It is important to note that the level of optimality is not equal to relative abundance of cells, but rather reflects the strategy adopted to optimize the biomass yield. We observed that interspecies hydrogen transfer occurred in addition to DIET whenever the optimality levels of the electron-accepting organism was at least 1.8 times that of the electron-donating organism ( Fig. 5b ). In other words, when interspecies hydrogen transfer was modelled in silico to occur along with DIET, G. sulfurreducens tends to adopt a strategy that is relatively more optimal. In a scenario where the relative optimality levels of the two organisms are of similar orders of magnitude, it is predicted that the energetic requirements of G. metallireducens preclude the possibility of interspecies hydrogen transfer. This is largely due to the energetic advantage conferred to the electron-donating organism due to the proton gradient established during DIET compared with interspecies hydrogen transfer ( Supplementary Fig. S4 ). To further explore other environmental factors that could determine the preference of DIET as the mode of electron exchange, we performed a sensitivity analysis. We found the proton intake flux by the partner accepting electrons ( G. sulfurreducens ) as the critical factor that affects the efficiency of DIET ( Supplementary Fig. S5 ). Although the proton intake flux had no impact on the energy efficiency during interspecies hydrogen transfer, it had a linear effect on the energy yield in DIET and DIET+acetate transfer. Hence, a combination of genomic characteristics, environmental factors such as proton availability in the local microenvironment and aspects of community dynamics like relative optimality of electron acceptor and donor organisms are expected to have a role in determining the preference of interspecies electron transfer mechanisms. Microorganisms engage in diverse partnerships and complex interactions in their natural environment. The extent and nature of these partnerships have a crucial role in the global cycling of nutrients and energy. Syntrophic associations between microorganisms are dominant mediators of all the major biogeochemical cycles in anoxic environments [2] , [3] , [4] . The obligate nature of most of these associations necessitate a tight coupling of the metabolism and energetics, typically resulting in the formation of compact aggregates that operate at thermodynamic equilibrium [1] . Despite the rapid development of high-throughput sequencing and metagenomic technologies, almost all modelling approaches used to study these interspecies interactions have been limited to characterizing the metabolic exchanges between the constituents without accounting for the functional effect of the potentially different mechanisms of reducing equivalent transfer. Here, for the first time, we present a multi-omic modelling workflow to investigate metabolic dynamics and mechanisms of electron flow in the laboratory evolved syntrophic coculture of G. metallireducens and G. sulfurreducens at three distinct levels of complexity. Reconstruction of the energetics associated with extracellular electron transfer pathways enabled the mechanistic basis of investigation of the relative efficiencies of DIET versus other alternatives. In the syntrophic association of G. metallireducens and G. sulfurreducens , the model predictions reaffirmed the prevalence of DIET as the mode of electron exchange. The reactions essential for the maintenance of this syntrophic association exclusively corresponded to those involved in DIET. The energetic efficiency of DIET was predicted to be directly impacted by the proton influx, unlike the case of interspecies hydrogen transfer. This study further presents a comparative analysis of the factors that determine the preference of DIET or interspecies hydrogen transfer. This is demonstrated by analysing a similar system of syntrophic ethanol oxidation involving P. carbinolicus and G. sulfurreducens . This revealed that metabolic features such as energy conservation via proton gradient or substrate-level phosphorylation, environmental factors such as proton availability in the local microenvironment, and microbial community dynamics could have a role in deploying DIET or interspecies hydrogen transfer mechanisms during syntrophic associations. In addition to characterizing the syntrophy at the level of metabolites and electron flow, our integration of transcriptomic and physiological data with genome-scale models enabled us to describe the interplay between the mechanisms of electron flow. By modelling genetic perturbations that eliminated additional electron transfer via acetate, we arrived at the positive effect of acetate transfer on DIET. We demonstrated that in the absence of acetate transfer, the efficiency of DIET is suboptimal. The ability to extract such interaction motifs is of particular importance when studying complex microbial communities where multiple mechanisms of electron exchange are likely to be prevalent. It is possible that other syntrophic consortia will exploit a similar synergy of different electron flow mechanisms in a condition-dependent manner. The knowledge of such unique interaction motifs between modes of electron transfer will have a significant impact on the design of synthetic syntrophic consortia for several bioengineering applications in the future [39] . Finally, we obtained novel insights into the dynamics of interaction and adaptive responses to syntrophic growth. Two distinct phases of syntrophic growth characterized by maximal and suboptimal electron transfer were observed. As the electron transfer scenario transitioned from suboptimal to maximal (Phase B to A), the relative abundance of G. sulfurreducens increased. This led us to postulate that G. sulfurreducens actively drives the association by dominating the interaction dynamics. This inference was found to be consistent with a previous finding that the beneficial mutation that promoted syntrophic association was in G. sulfurreducens . In other words, the organism that relies on the electrons transferred ( G. sulfurreducens ) from its partner had the need to actively respond to the selection pressure by undergoing changes at the genomic level. However, the partner that provides electrons ( G. metallireducens ) seemed to respond only at the level of the transcriptome. This type of dynamics could have several evolutionary implications, suggesting that in syntrophic associations, the accepting partner streamlines its metabolic capabilities to enhance the most efficient mode of electron transfer. This could be of particular relevance when characterizing methanogenic consortia. Given that methanogens are typically involved in syntrophic relationships, it is possible that they respond similarly to the availability of the electron donor by streamlining their metabolic capabilities for the most efficient utilization strategy. In fact, a recent study on the functional response of M. maripaludis to syntrophic growth in association with D. vulgaris revealed that, the methanogen uses paralogous genes to adapt to the changing substrate availability when growing syntrophically compared with growing as a monoculture [40] . An approach like the one presented here, that integrates genome resequencing, metatranscriptomics and genome-scale modelling, would likely allow for a deeper mechanistic insight into the dynamics and adaptation of the syntrophic interaction of M. maripaludis and D. vulgaris . In summary, this study represents a multi-omic approach to elucidate the electron transfer mechanism and to characterize the metabolic phenotype of a syntrophic consortium at multiple levels of complexity. This integrated approach demonstrates that energetic limits due to obligate syntrophic associations are reflected in the genome and the transcriptome of the microorganisms, thereby providing a comprehensive alternative framework for detailed mechanistic characterization. As the approach developed here is modular, it can be easily extended for the characterization of other complex communities. The models being developed in these studies will be important for understanding the functioning of anaerobic microbial communities and could aid in predicting the influence of environmental changes on methane emissions and other aspects of the carbon cycle. Reconstructing a genome-scale model of syntrophy To model the syntrophy between G. metallireducens and G. sulfurreducens , the existing genome-scale metabolic reconstructions of the two species were updated and expanded. A comparative reconciliatory process involving automated reconstructions from MODEL SEED [41] , draft reconstruction based on the updated genome annotation, existing reconstruction and extensive manual curation was used to update and expand the metabolic model of G. metallireducens . This updated model was used to expand the genome-scale metabolic model of G. sulfurreducens. Homologues to G. sulfurreducens genes were identified in the G. metallireducens genome using a bi-directional Smith-Waterman alignment. A 60% ID cutoff was used to identify the homologues. The most recent updated annotation (AE017180 version 2) of G. sulfurreducens was then used to curate the homology matches. A distinct periplasmic compartment was also incorporated into the model. This procedure also included the explicit reconstruction of the extracellular electron transfer pathways as described in Fig. 1a . Specifically, the redox potentials for the thermodynamic analysis on the various redox couples were obtained from Thauer et al. [42] The proton translocation stoichiometry was approximated using the theoretical limits described in ref. 43 . While the exact mechanistic aspects of extracellular electron transfer remains to be characterized, this thermodynamic consistency allows us to model the energetic requirements of electron transfer. The two genome-scale reconstructions were integrated into a combined model by extending the compartmentalized framework. A compartment called the SMP was introduced. This compartment was meant to facilitate the exchange of metabolites between the two genome-scale models as well as their interaction with the extracellular environment. To achieve this, the outer membrane transporters in each of the genome-scale models were replaced by transporters that facilitated transfer from the respective periplasmic compartments to the SMP. Exchange reactions were added for all metabolites present in the SMP ( Supplementary Fig. S6 ). Modelling DIET DIET was accounted for by introducing a reaction that represents stoichiometric transfer of electrons between the outer membrane cytochromes of the two Geobacter species. The flux through this reaction was constrained based on the midpoint potential of OmcS, an outer membrane cytochrome of G. sulfurreducens . The maximum electron transfer flux through DIET was calculated by scaling the midpoint potential of OmcS ( E omcS ) using the equation In this equation, E Fe(III)citrate represents the midpoint potential of Fe(III) citrate and Y Fe/EtOH represents the ratio of Fe(III) reduction rate to the oxidation rate of the electron donor (ethanol). Physiological data measurements and growth conditions All growth experiments of G. metallireducens and G. sulfurreducens (WT and CS K.O. strains) were performed using strict anaerobic culturing techniques. Cultures were incubated in 160 ml serum bottles sealed with butyl rubber stoppers and filled with 100 ml of media. The culture medium was provided with 40 mM fumarate and 20 mM ethanol as the sole electron donor as described [20] . For determination of substrate depletion and metabolite production, samples were withdrawn under strict anaerobic conditions with hypodermic needles and syringes. Samples were passed through 0.2 m Acrodisc filters and were diluted before analysis. Changes in ethanol concentration over time were monitored by gas chromatograph equipped with a headspace sampler and a flame ionization detector (Clarus 600; PerkinElmer, California) [17] . Changes in concentration of volatile fatty acids, such as fumarate, succinate, malate and acetate were determined by high performance liquid chromatography with a fast-acid column (Bio-Rad, Hercules, CA) with an eluent of 8 mM H 2 SO4 and UV detection at 210 nm. Cell biomass increase over time was determined in four replicate cocultures (100 ml each) of G. metallireducens with G. sulfurreducens (WT and CS K.O. strains). Aggregates were collected at different growth stages by centrifuging for 15 min at 3600 g , washed in isotonic buffer, and pelleted at 3600 g The pelleted cell suspensions were freeze dried for 48 h on a Labconco lyophilizer. Dry mass was weighed before re-suspension in 0.5% SDS for determination of total protein content using the bicinchoninic acid method [44] with a protein standard. Simulating syntrophic growth using the genome-scale model The genome-scale metabolic reconstruction of the syntrophic association was represented in a mathematical format in the form a stoichiometric matrix (S). The rows of the matrix represent the metabolites in the network, while the columns represent the reactions. Flux balance analysis, where the flux through a particular objective reaction is optimized subject to a set of constraints, was used to characterize the system [45] . In this particular case, the objective of the optimization was maximizing the flux through the biomass objective functions of both G. metallireducens and G. sulfurreducens . The relative abundance of the two species was calculated by determining the ratio of the fluxes through the biomass objective functions of the respective organisms [13] . Typically, the constraints for the optimization problem include upper and lower bounds (ub, lb) for reaction fluxes calculated from thermodynamic and enzyme kinetics. In this simulation, an additional constraint on the flux through DIET was applied based on . Constraints on ethanol, and fumarate uptake rates were applied based on experimentally measured physiological rates. All ions, and water were allowed to enter the network freely. Additionally, the loopless COBRA constraint was applied to eliminate thermodynamically infeasible loops from the solution [46] . Reaction deletion analysis and phenotype phase plane analysis were carried out using the singleRxnDeletion and phenotypePhaseplane functions in the COBRA toolbox [47] . The genome-scale model of syntrophy is available as Supplementary Data 3 and can be used in the COBRA toolbox. Monte Carlo sampling and differential reaction activity Monte Carlo sampling was applied on the integrated genome-scale model of the syntrophic consortium to generate a set of uniform, feasible flux distributions. A modified version of the artificially centred hit and run algorithm called gpSampler [47] , [48] was implemented to sample both the WT and CS K.O strains. Differential reaction activity was computed based on the sampled flux distributions as done in a previous study [49] , [50] . Significance of change was determined at a false discovery rate of 0.05 [51] . Using the gene–protein reaction associations in the genome-scale model, the genes corresponding to the reactions showing differential activity were obtained. This was compared with the list of differentially expressed genes obtained from transcriptomic profiling using RNA-seq. Trasnscriptomic profiling of the aggregates using RNA-seq Total RNA was isolated from wild type and mutant aggregates using the acid phenol method [52] , [53] . Residual DNA was removed with a 30 min DNAse I digestion at 37 °C (Qiagen) followed by purification with the RNeasy Mini kit (Qiagen). A total of 2.5 μg of total RNA was treated with the gram-negative RiboZero kit (Epicentre). Paired end, strand-specific RNA sequencing was performed using a variation of the 2′-deoxyuridine, 5′-triphosphate dUTP method outlined in refs 54 , 55 with the following changes. Hundred nanograms of rRNA subtracted RNA was fragmented with RNA fragmentation reagents (Ambion) for 3 min at 70 °C. First-strand synthesis was primed using random hexamers (Invitrogen). Paired-end libraries were created for Illumina sequencing using Illumina compatible adapters, which were ligated onto the double-stranded cDNA fragments [56] . Library amplification was monitored using quantitative polymerase chain reaction, and the reactions were stopped just as libraries entered exponential amplification. Final libraries were purified with 1.0 × AMPure XP Beads (Beckman Coulter quantified using the 2100 Bioanalyzer (Agilent) and sequenced on an Illumina GAIIx. Transcriptomic data is available from EMBL database at accession codes ERP001972 and ERP001975. Transcript quantification The obtained RNA-seq reads were aligned to the concatenated genome sequences of G. metallireducens and G. sulfurreducens (RefSeq accession codes NC_007517.1 and NC_002939) using the short-read aligner Bowtie [57] with two mismatches allowed per read alignment. To estimate transcript abundances, FPKM values were calculated using the tool Cufflinks ( http://www.cufflinks.cbcb.umd.edu/ ) [58] with appropriate parameters set for the strand-specific library type and upper-quartile normalization. Differential expression analysis was carried out using cuffdiff, with upper-quartile normalization and appropriate parameters set for strand-specific library type. A fold change of greater than twofold and false discovery rate cutoff of 0.05 was used to determine significant differential expression between two different conditions. Functional enrichment analysis To determine if the differentially expressed genes were enriched for any particular metabolic subsystem in the genome-scale model, a hypergeometric test was performed using the hygecdf function in MATLAB. A P -value cutoff of 0.05 was used to determine significance. Resequencing and mutation identification Nine parallel replicate cocultures of G. metallireducens and G. sulfurreducens were sequenced after 780 generations using Illumina sequencing and the resulting mutations were compared to those identified after 100 generations [20] . The concatenated genomes of G. metallireducens (NC_007517) and G. sulfurreducens (AE017180 version 2) were used as the reference for mutation identification. Illumina reads from the nine different resequencing experiments were iteratively aligned to this reference using MosaikAligner (Stromberg and Marth http://bioinformatics.bc.edu/marthlab/Mosaik ). The number of allowed mismatches in the alignment was increased from 0–5 in each iterations with the unaligned reads used as the input for the subsequent iteration. The alignments were processed using a custom script written in-house (described in ref. 59 ) to obtain the fold coverage at single base-pair resolution. A coverage cutoff of 10 × was employed for SNP identification and lack of coverage was used to identify deletion. Furthermore, a particular location was deemed polymorphic in each of the nine experiments, if the observed nucleotide count was greater than twice the count of the actual nucleotide in the reference sequence at that position. Finally, a particular location was considered to be a mutation, if it was found in at least seven of the nine replicates. Accession codes: The transcriptomic data have been deposited in the EMBL database under accession codes ERP001972 and ERP001975 . How to cite this article: Nagarajan, H. et al. Characterization and modelling of interspecies electron transfer mechanisms and microbial community dynamics of a syntrophic association. Nat. Commun. 4:2809 doi: 10.1038/ncomms3809 (2013).